UNR facilitates the interaction of MLE with the lncRNAroX2duringDrosophiladosage compensation Dosage compensation is a regulatory process that balances the expression of X-chromosomal genes between males (XY) and females (XX). In Drosophila, this requires non-coding RNAs and RNA-binding proteins (RBPs) whose specific functions remain elusive. Here we show that the Drosophila RBP UNR promotes the targeting of the activating male-specific-lethal complex to the X-chromosome by facilitating the interaction of two crucial subunits: the RNA helicase MLE and the long non-coding RNA roX2 . In Drosophila , dosage compensation involves the binding of the MSL dosage compensation complex (MSL–DCC) to hundreds of sites on the single male X-chromosome and the subsequent twofold hypertranscription of active genes [1] . The MSL–DCC contains five proteins: MSL1, MSL2, MSL3, Maleless (MLE) and Males-absent-on-first (MOF), and two long non-coding RNAs, RNA on X ( roX ) 1 and 2 , which differ in size and sequence but display redundant functions [2] . MSL2 is the limiting subunit of the MSL–DCC and, together with MSL1, nucleates complex formation at specific X-chromosomal sites known as high-affinity sites (HAS) [3] , [4] . The RNA helicase MLE colocalizes with MSL2 at HAS and facilitates the incorporation of roX into the complex. The RNA is important for the distribution of the MSL–DCC along the X-chromosome, where it activates target genes [2] , [5] , [6] , [7] . Upstream of N-Ras (UNR) is a conserved RNA-binding protein (RBP) containing five cold-shock domains (CSD) that regulates mRNA translation and stability by interacting with single-stranded RNA [8] . We previously showed that Drosophila UNR performs sex-specific opposing roles in dosage compensation. In females, UNR inhibits MSL–DCC assembly by repressing the synthesis of MSL2 (ref. 9 ). In males, UNR promotes the targeting of the MSL–DCC to the X-chromosome by a poorly understood mechanism that does not involve translational regulation of MSL proteins [10] . UNR-dependent regulation can be recapitulated in male S2 cells, which express only roX2 (ref. 11 ). In this work we describe our efforts to determine whether UNR interacts with the DCC assembly and targeting machinery in more specific ways. Primed by the finding of a preferred RNA-binding element for UNR close to the known roX remodelling site of the helicase MLE [12] , we systematically explored the relationship between UNR and MLE. We found that UNR facilitates the binding of MLE to its target at limiting MLE concentrations. These biochemical analyses approximate the physiological conditions to a good extent, since depletion of UNR also diminishes the MLE– roX interaction and reduces the association of MLE with HAS in dosage-compensating cells. These results identify UNR as a general RBP with specific roles in dosage compensation. Direct binding of UNR to roX2 stem–loops To assess whether recombinant UNR could directly bind to roX2 , we employed an electrophoretic mobility shift assay (EMSA). UNR bound full-length roX2 RNA (not shown) and several roX2- derived fragments ( Fig. 1 ). UNR interacted most strongly with a roX2 fragment spanning nucleotides 316–379 ( Fig. 1b , fragment E). Interestingly, this purine-rich region is located within stem–loop 6 (SL6) just upstream of a prominent, conserved stem–loop structure (SLroX2 or SL7) [12] that, when multimerized, is sufficient to restore the X-chromosomal targeting defects of a roX null mutant [13] . Pull-down assays using MS2-tagged RNA as bait confirmed that UNR bound with highest affinity to roX2 fragments containing SL6 ( Fig. 1c ). 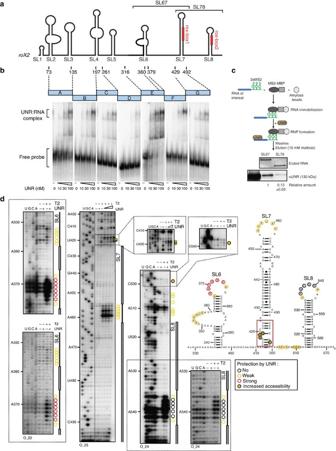Figure 1: UNR binds toroX2directly. (a) Schematic representation ofroX2and derivatives. The stem–loops (SL), the roX boxes and the limits ofroX2A–G fragments are indicated. (b) Analysis of UNR binding toroX2fragments by EMSA. (c) Analysis of UNR binding to SLs in the 3′ half ofroX2by RNA pulldown. Three copies of MS2 coat protein-binding sites (MS2) fused to the RNA of interest are recognized by MBP-tagged MS2 coat protein, which in turn binds to amylose beads. After adding recombinant UNR, RNPs are washed and eluted. Quantifications correspond to the average of UNR binding in three experiments. Full-size blots corresponding to this Figure are shown inSupplementary Fig. 5. (d) Footprinting of UNR on full-lengthroX2treated with RNase T2. cDNAs obtained by primer extension were electrophoretically separated. Lanes labelled U, G, C, A represent Sanger sequencing ladders. Nucleotides are numbered relative to nucleotide +1 ofroX2. Protected nucleotides are labelled with open circles (black, yellow and red for no, weak and strong protections, respectively) and nucleotides that gain accessibility upon UNR binding are indicated with filled circles. The region of SL7 potentially remodelled by UNR is indicated by a red square. A schematic summary of the experimental footprinting data is shown on the right. The insets show independent experiments at higher resolution, or different exposures of the same gel. Figure 1: UNR binds to roX2 directly. ( a ) Schematic representation of roX2 and derivatives. The stem–loops (SL), the roX boxes and the limits of roX2 A–G fragments are indicated. ( b ) Analysis of UNR binding to roX2 fragments by EMSA. ( c ) Analysis of UNR binding to SLs in the 3′ half of roX2 by RNA pulldown. Three copies of MS2 coat protein-binding sites (MS2) fused to the RNA of interest are recognized by MBP-tagged MS2 coat protein, which in turn binds to amylose beads. After adding recombinant UNR, RNPs are washed and eluted. Quantifications correspond to the average of UNR binding in three experiments. Full-size blots corresponding to this Figure are shown in Supplementary Fig. 5 . ( d ) Footprinting of UNR on full-length roX2 treated with RNase T2. cDNAs obtained by primer extension were electrophoretically separated. Lanes labelled U, G, C, A represent Sanger sequencing ladders. Nucleotides are numbered relative to nucleotide +1 of roX2 . Protected nucleotides are labelled with open circles (black, yellow and red for no, weak and strong protections, respectively) and nucleotides that gain accessibility upon UNR binding are indicated with filled circles. The region of SL7 potentially remodelled by UNR is indicated by a red square. A schematic summary of the experimental footprinting data is shown on the right. The insets show independent experiments at higher resolution, or different exposures of the same gel. Full size image Because of the roles of UNR in RNA metabolism, we next assessed whether UNR binding affected roX2 levels, nucleocytoplasmic distribution or splicing of its major isoforms in S2 cells. UNR depletion showed no effect on any of these features ( Supplementary Fig. 1 ). To gain insight into UNR– roX2 interactions, we performed enzymatic and chemical footprinting ( Fig. 1d and Supplementary Fig. 2 ). Addition of UNR protected unpaired nucleotides of SL6, in particular the terminal loop (nts 367–374) and the internal bulge (nts 352–357), suggesting UNR binding to these regions. UNR also protected to a lower extent the terminal loop of SL7 and the single-stranded region between SL7 and SL8 but did not protect efficiently the terminal loop of SL8. These results confirmed that UNR interacts preferentially with SL6. Mutational analysis showed that UNR recognizes the purine-rich stretches in the loops ( Supplementary Fig. 3 ). Interestingly, nucleotides 417–419 and 497 were rendered more reactive upon the addition of UNR. These positions form a 7 bp-extended version of SL7 ( Fig. 1d ), which maybe disrupted by UNR. These results suggest a role for UNR as a roX2 chaperone. UNR interacts with MLE in a roX2 -dependent manner In bacteria, CSD-containing RNA chaperones associate with RNA helicases to promote RNA remodelling [14] . We, thus, asked whether UNR interacts with the RNA helicase MLE. Co-immunoprecipitation experiments with recombinant proteins demonstrated a weak interaction between MLE and UNR ( Fig. 2a , lane 3). Interestingly, this interaction was strongly stimulated by roX2 but not by an unrelated control RNA of similar length (compare lanes 3, 4 and 7). The interaction persisted after efficient RNase treatment, monitored by measuring the presence of trace-labelled roX2 in the pellet (lanes 3–5), indicating that roX2 promotes strong direct interactions between MLE and UNR, or that any connecting RNA within the complex is protected from RNase digestion. To test whether these interactions occurred in vivo , we immunoprecipitated UNR from nuclear extracts of S2 cells. Although UNR is primarily cytoplasmic, a small amount can be found in the nucleus that interacts with MLE, but not with MSL3, indicating that the interaction is specific ( Fig. 2b , upper panel). Consistent with the in vitro data and with the presence of roX2 in the nucleus, the interaction of endogenous MLE and UNR is resistant to RNase treatment after formaldehyde crosslinking, suggesting that interactions involve protein–protein crosslinks and not merely protein–RNA crosslinks ( Fig. 2b , lower panel). Altogether, the data suggest that UNR, MLE and roX2 form a complex. Indeed, a ternary complex is detected by EMSA when roX2 or its 3′ half fragment (SL678) is incubated with recombinant UNR and MLE ( Supplementary Fig. 4 ). 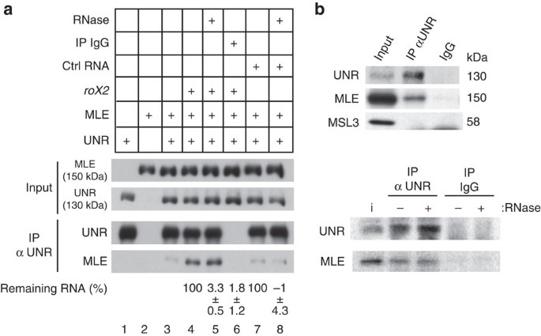Figure 2: UNR interacts with MLE. (a) The interaction of UNR and MLE is direct and stimulated byroX2. Recombinant UNR, MLE and/or trace-labelledroX2SL678 or a control RNA of similar size corresponding to the 3′-UTR ofTollwere mixed in equimolar amounts, UNR was immunoprecipitated and MLE assessed by western blot analysis after optional incubation with RNases A+T1 followed by extensive washing. Nonspecific IgGs were used as negative control. The RNA remaining in the pellet was quantified and normalized to that in the absence of RNase. Quantifications represent the average of two experiments. (b) Interaction of the endogenous proteins. Nuclear extracts were obtained from formaldehyde-crosslinked nuclei and used to immunoprecipitate UNR. Similar reactions with nonspecific IgGs served as controls. The presence of MLE and MSL3 in the pellet was assessed by with western blot analysis. In some reactions the pellet was treated with RNases A+ T1 (lower panel). Full-size blots corresponding to this Figure are shown inSupplementary Fig. 5. Figure 2: UNR interacts with MLE. ( a ) The interaction of UNR and MLE is direct and stimulated by roX2 . Recombinant UNR, MLE and/or trace-labelled roX2 SL678 or a control RNA of similar size corresponding to the 3′-UTR of Toll were mixed in equimolar amounts, UNR was immunoprecipitated and MLE assessed by western blot analysis after optional incubation with RNases A+T1 followed by extensive washing. Nonspecific IgGs were used as negative control. The RNA remaining in the pellet was quantified and normalized to that in the absence of RNase. Quantifications represent the average of two experiments. ( b ) Interaction of the endogenous proteins. Nuclear extracts were obtained from formaldehyde-crosslinked nuclei and used to immunoprecipitate UNR. Similar reactions with nonspecific IgGs served as controls. The presence of MLE and MSL3 in the pellet was assessed by with western blot analysis. In some reactions the pellet was treated with RNases A+ T1 (lower panel). Full-size blots corresponding to this Figure are shown in Supplementary Fig. 5 . Full size image UNR promotes the interaction of MLE with roX2 in vitro Intriguingly, the base of the extended SL7 of roX2 that is potentially remodelled by UNR (see box in Fig. 1d ) serves as a binding site for MLE, which disrupts SL7 thereby promoting subsequent interactions with MSL2 (ref. 12 ). Thus, melting of the base of SL7 by UNR and exposure of the corresponding nucleotides could facilitate MLE interaction with roX2 . To test this hypothesis, we first monitored the binding of recombinant UNR and MLE to roX2 derivatives using RNA pull-down assays ( Fig. 3 ). We first titrated MLE on SL67 in the presence or absence of UNR. At high concentrations, MLE was able to bind SL67 ( Fig. 3b , lane 5). MLE, however, was unable to efficiently bind the target RNA at reduced concentrations ( Fig. 3b , lanes 2–4). Remarkably, under those conditions the interaction of MLE with SL67 was strongly facilitated by adjacent UNR binding ( Fig. 3b , compare lanes 4 and 8). To test the correlation between MLE and UNR binding, we employed the roX2 derivatives SL2345 and SL67. UNR bound to both RNAs in the absence of MLE and, consistent with the EMSA ( Fig. 1b ), it bound with higher affinity to SL67 ( Fig. 3c ). MLE bound to roX2 fragments after UNR addition in a manner that correlated with the strength of UNR binding ( Fig. 3c , lanes 3 and 6). In addition, MLE bound strongly to full-length roX2 in the presence of UNR, and this binding was reduced upon deletion of either SL6 or SL7 ( Fig. 3d , compare lane 8 with lanes 9 and 10). These results indicate that UNR promotes the association of MLE with roX2 in vitro . 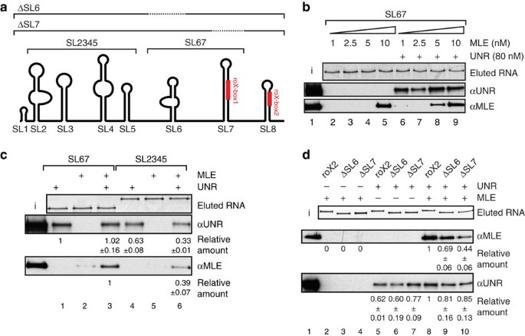Figure 3: UNR facilitates the interaction of MLE withroX2 in vitro. (a) Schematic representation ofroX2and derivatives used for RNA pulldown. (b) Titration of MLE in the presence or absence of UNR. MS2-tagged SL67 RNA was immobilized on amylose beads and incubated with MLE and UNR. Complexes were eluted as described in the Methods section. The effect of UNR on MLE binding torox2is visible at low MLE concentrations. (c) Correlation between UNR and MLE binding. MS2-tagged SL67 and SL2345 were used for RNA pulldown in the presence of MLE and/or UNR, and complexes were eluted. Bound MLE and UNR were quantified relative to the amount of eluted RNA, and normalized to the value obtained for SL67. Quantifications correspond to the average of two independent experiments. (d) UNR promotes the binding of MLE to full-lengthroX2. UNR and MLE were allowed to bind to full-length, ΔSL6 and ΔSL7roX2RNAs, and the RNPs were eluted. The percentage of bound UNR and MLE was quantified relative to the amount of eluted RNA. Values were normalized to MLE and UNR binding to full-lengthroX2. s.d.’s were determined from three independent experiments. Full-size blots corresponding to this Figure are shown inSupplementary Fig. 6. Figure 3: UNR facilitates the interaction of MLE with roX2 in vitro . ( a ) Schematic representation of roX2 and derivatives used for RNA pulldown. ( b ) Titration of MLE in the presence or absence of UNR. MS2-tagged SL67 RNA was immobilized on amylose beads and incubated with MLE and UNR. Complexes were eluted as described in the Methods section. The effect of UNR on MLE binding to rox2 is visible at low MLE concentrations. ( c ) Correlation between UNR and MLE binding. MS2-tagged SL67 and SL2345 were used for RNA pulldown in the presence of MLE and/or UNR, and complexes were eluted. Bound MLE and UNR were quantified relative to the amount of eluted RNA, and normalized to the value obtained for SL67. Quantifications correspond to the average of two independent experiments. ( d ) UNR promotes the binding of MLE to full-length roX2 . UNR and MLE were allowed to bind to full-length, ΔSL6 and ΔSL7 roX2 RNAs, and the RNPs were eluted. The percentage of bound UNR and MLE was quantified relative to the amount of eluted RNA. Values were normalized to MLE and UNR binding to full-length roX2 . s.d.’s were determined from three independent experiments. Full-size blots corresponding to this Figure are shown in Supplementary Fig. 6 . Full size image UNR promotes the interaction of MLE with roX2 in vivo To test whether UNR promotes the association of MLE with roX2 in vivo , we depleted UNR from S2 cells. Ablation of UNR diminished the amounts of roX2 associated with the endogenous helicase ( Fig. 4a , right panel). This effect could neither be attributed to variations in the amounts of MLE or roX2 upon UNR depletion nor to differences in the efficiency of MLE immunoprecipitation ( Fig. 4a , middle and left panels). To explore whether the reduced MLE– roX2 interaction affects the association of MLE with its chromosomal targets, the HAS, we employed chromatin immunoprecipitation (ChIP). Notably, we found that UNR depletion decreased the MLE association to four different HAS ( Fig. 4b , left panel). As controls, UNR depletion did not affect the association of MLE to promoters within the same genes ( Fig. 4b ), or the association of MOF to HAS or to an autosomal gene ( Fig. 4b , right panel). Altogether, these results demonstrate a role for UNR in facilitating the binding of the RNA helicase MLE with its target sites on roX2 RNA in vitro and in vivo . 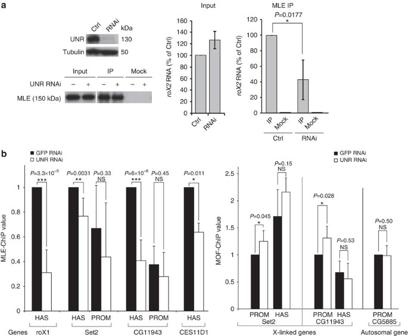Figure 4: UNR facilitates the interaction of MLE withroX2 in vivo. (a) Nuclear extracts from S2 cells depleted of UNR (+, RNA interference (RNAi)) or GFP (−, Ctrl) were used to immunoprecipitate MLE (IP), carrying empty beads as control (mock). The amount ofroX2associated to MLE was determined with RT–qPCR, and values were normalized to MLE binding in control RNAi cells (right panel). Error bars represent the s.d. of six experiments. The efficiency of UNR immunodepletion and MLE immunoprecipitation was assessed using western blot analysis (left panels), and the levels of inputroX2were monitored with RT–qPCR (middle panel). Full-size blots corresponding to this Figure are shown inSupplementary Fig. 6. (b) Left panel, UNR promotes MLE binding to HAS. Binding of MLE toSet2,CG11943,roX1and CES11D1 HAS was measured using ChIP in control (GFP) or UNR-depleted cells. Amplification of nearby regions within the same genes was carried out as internal control and used for correction. Values represent the ChIP/input ratio normalized to the GFP control. The binding of MLE to promoters was assessed as negative control. The average of at least four independent experiments is shown. Right panel, UNR does not affect the genomic localization of MOF. Binding of MOF toSet2,CG11943andCG5885HAS and/or promoters in control (GFP) or UNR-depleted cells, measured as described above. The average of at least three independent experiments is shown. Asterisks indicate level of statistical significance using the Student’st-test (*P<0.05; **P<0.005; ***P<0.001). Figure 4: UNR facilitates the interaction of MLE with roX2 in vivo . ( a ) Nuclear extracts from S2 cells depleted of UNR (+, RNA interference (RNAi)) or GFP (−, Ctrl) were used to immunoprecipitate MLE (IP), carrying empty beads as control (mock). The amount of roX2 associated to MLE was determined with RT–qPCR, and values were normalized to MLE binding in control RNAi cells (right panel). Error bars represent the s.d. of six experiments. The efficiency of UNR immunodepletion and MLE immunoprecipitation was assessed using western blot analysis (left panels), and the levels of input roX2 were monitored with RT–qPCR (middle panel). Full-size blots corresponding to this Figure are shown in Supplementary Fig. 6 . ( b ) Left panel, UNR promotes MLE binding to HAS. Binding of MLE to Set2 , CG11943 , roX1 and CES11D1 HAS was measured using ChIP in control (GFP) or UNR-depleted cells. Amplification of nearby regions within the same genes was carried out as internal control and used for correction. Values represent the ChIP/input ratio normalized to the GFP control. The binding of MLE to promoters was assessed as negative control. The average of at least four independent experiments is shown. Right panel, UNR does not affect the genomic localization of MOF. Binding of MOF to Set2 , CG11943 and CG5885 HAS and/or promoters in control (GFP) or UNR-depleted cells, measured as described above. The average of at least three independent experiments is shown. Asterisks indicate level of statistical significance using the Student’s t -test (* P <0.05; ** P <0.005; *** P <0.001). Full size image The incorporation of roX RNA into the MSL–DCC is crucial for dosage compensation. In the absence of MLE (and roX ), MSL2 and MSL1 can associate with HAS but no functional DCC is assembled that distributes the activating histone acetylation to the target genes [15] , [16] , [17] . ChIP experiments show prominent, specific interaction of MLE at HAS in S2 cells [6] . Our current data now suggest that the general RBP UNR facilitates this interaction. Remarkably, UNR also binds and regulates the activity of msl2 mRNA together with the sex determination switch SXL [9] , [18] , suggesting that sex determination and dosage compensation have co-evolved to employ similar factors from the large portfolio of RBPs. UNR, thus, extends the small list of RBPs involved in dosage compensation. Such factors include hnRNPU and YY1, which tether the lncRNA Xist to the inactive X-chromosome during mammalian dosage compensation [19] , [20] . Rather than a molecular tether, however, the role of UNR seems more transient and directed to facilitate initial steps of MSL–DCC assembly through the modulation of RNA conformation. UNR, therefore, acts as a ‘catalyst’ of the MLE– roX interaction. RNA structural transitions are at the basis of many fundamental post-transcriptional processes [21] . Our results illustrate the emerging concept that lncRNA structural dynamics may contribute to chromatin organization, and indicate that general RBPs, such as UNR, can be harnessed to contribute key molecular events in the assembly of specialized machineries. Cell culture and RNA interference treatment Cells were maintained at 25 °C in Schneider’s Medium (GIBCO) supplemented with 1.2 mM L -glutamine (GIBCO), 1% (v/v) penicilin/streptomycin (GIBCO) and 10% fetal bovine serum (FBS; Invitrogen). For RNA interference treatment, 1.5 × 10 6 cells were incubated with 15 μg of dsRNA corresponding to the UNR-coding region (nt 2139–2691 relative to the start codon) or with dsRNAs against green-fluorescent protein (GFP) as control. Cells were recovered 6 days after plating and the efficiency of UNR depletion was monitored with western blot using anti-UNR [7] and anti-tubulin (Sigma) antibodies. Quantitative RT–PCR Total RNA from control and UNR-depleted S2 cells was extracted using Trizol and treated with Turbo DNAse (Ambion). First-strand cDNAs were synthesized from 500 ng of total RNA with Superscript II (Invitrogen). Parallel samples without reverse transcriptase were carried as control. The reaction mixture was diluted and roX2 was amplified using quantitative PCR using the Power SYBR Green kit (Applied Biosystem). Quantitive PCR (qPCR) was performed on an Applied Biosystem device and analysed using the associated software. Quantitative values were normalized to the internal standard actin (oligonucleotides are detailed in Supplementary Table 1 ). Subcellular fractionation and northern blot Nucleocytoplasmic fractionation was performed by resuspending cells in hypotonic buffer (10 mM HEPES pH 7.6, 10 mM K-Acetate, 0.5 mM Mg-Acetate, 0.5% Triton X-100, 5 mM dithiothreitol (DTT), 1 × protease inhibitor cocktail from Roche). Cells were incubated on ice for 5 min, centrifuged and the supernatant recovered as the cytoplasmic fraction. Nuclear pellets were washed with phosphate-buffered saline (PBS), and RNA was extracted from the nuclear and cytoplasmic fractions using Trizol. For northern blot analysis of roX2 subcellular localization, 10 μg of total RNA, 2 μg of nuclear RNA and an amount of cytoplasmic RNA proportional in volume to the nuclear fraction were resolved in a 2.5% denaturing agarose gel, transferred and hybridized to antisense-labelled oligonucleotides ( Supplementary Table 1 ). Northern blot of roX2 transcript isoforms was performed on 25 μg of total RNA using a random-primed probe against roX2 isoform C. Immunoprecipitation and western blot UNR was immunoprecipitated from S2 nuclear extracts prepared as follows. S2 nuclei were resuspended in PBS and crosslinked with 0.5% formaldehyde at room temperature for 10 min. Crosslinking was quenched by the addition of 125 mM glycine. Nuclei were washed with PBS and proteins were extracted with RIPA buffer (150 mM NaCl, 10 mM TRIS pH 7.5, 0.1% SDS, 1% deoxycholate, 5 mM EDTA, 1% Triton X-100, 1 × protease inhibitor cocktail from Roche) after incubation for 20 min on ice, and sonicated using a bioruptor sonicator (high power, 30 s ON/30 s OFF, 6 min total). Purified custom-made [9] anti-UNR IgGs were bound to Protein A dynabeads (Invitrogen) and UNR immunoprecipitation was performed for 1 h at 4 °C. Beads were washed three times with 10 vol of 1XNET (50 mM TRIS-HCl pH 7.5, 150 mM NaCl, 0.1% NP40, 1 mM EDTA), optionally treated with RNase A+T1, and resuspended in SDS buffer. Western blots were performed with anti-UNR [9] , anti-MLE [22] and anti-MSL3 (ref. 6 ) antibodies at dilutions of 1:1,000, 1:2,000 and 1:1,000, respectively. MLE was immunoprecipitated from extracts obtained by resuspending nuclei in Triton X buffer (0.5 mM EDTA, 150 mM NaCl, 50 mM Tris–HCl pH 7.5, 1% Triton, 1 × protease inhibitor cocktail) and incubating the suspension for 1 h on ice. After immunoprecipitation, beads were divided into two aliquots, one for detection of MLE by western blot, the other for detection of roX2 after proteinase K elution followed by Trizol treatment and RT–qPCR. Before proteinase K elution, Firefly luciferase RNA was added as a spike-in control, and was used as a standard in the RT–qPCR analysis. U3 snoRNA was used to normalize the input samples. Firefly luciferase and U3 were detected using specific oligonucleotides ( Supplementary Table 1 ). For the experiment shown in Fig. 2a , recombinant UNR (10 nM) was incubated either alone or in the presence of equimolar amounts of recombinant MLE and trace-labelled roX2 SL678, or a control RNA of similar size corresponding to nucleotides 184–365 of Toll 3′-untranslated region (UTR). The mix was incubated for 30 min on ice in buffer D (20 mM Hepes pH 8.0, 20% glycerol, 0.2 mM EDTA, 1 mM DTT, 0.01% NP40) supplemented with 100 mM KCl and 150 ng μl −1 yeast tRNA and UNR immunoprecipitated as described above. After washes, beads were incubated with RNase A+T1 for 30 min at 37 °C and further washed. The presence of RNA in the pellet was monitored in a β-counter. RNA preparation and EMSA Radiolabelled roX2 RNA derivatives used in EMSA were prepared by in vitro transcription using hybridized oligonucleotide templates. One femptomole of RNA was mixed with increasing amounts of recombinant UNR in buffer D supplemented with 150 ng μl −1 tRNA and 100 mM KCl. The mix was incubated for 30 min on ice, and the complexes resolved in a native 4% acrylamide gel. Unlabelled roX2 RNAs were generated by run-off transcription (MEGAscript T7, Ambion) and purified via standard phenol:chloroform extraction followed by EtOH precipitation or with the RNeasy kit (Qiagen) according to manufacturer’s recommendations. Protein expression and purification His-FLAG-tagged, full-length UNR was purified according to the pET system user’s manual (Novagen). A second purification step using Flag columns was occasionally included. The protein was dialysed against buffer D. MS2–MBP was expressed in Escherichia coli . After cell sonication (Branson digital sonifier), MS2–MBP was purified on amylose beads and eluted in a buffer containing 10 mM maltose. The eluted fraction was then applied to a HiTrap Heparin column, and MS2–MBP was eluted by a linear gradient of 0–1 M NaCl in 10 mM sodium phosphate buffer. The protein was dialysed against buffer D and concentrated using an Amicon Ultra-4 column (Millipore) [23] . MLE was expressed in Sf21 cells using recombinant Baculoviruses expressing the wild-type protein fused to a C-terminal FLAG-tag. After Baculovirus infection for 3 days, harvested Sf21 cells were washed with ice-cold PBS, frozen in liquid nitrogen and stored at −80 °C. Sf21 cell pellets were resuspended on ice-cold Extraction Buffer EB (50 mM Hepes-KOH pH 7.6, 5% glycerol, 0.05% NP40, 0.5 mM EDTA, 1 mM MgCl 2 and protease inhibitor cocktail from Roche) containing 300 mM KCl (EB300). Twenty millilitres of EB300 were added to the cell pellet, sonicated (Branson digital sonifier) and centrifuged for 30 min at 30,000 g at 4 °C. The soluble protein fraction was incubated with equilibrated FLAG beads (anti-FLAG M2 Agarose, Sigma) for 3 h at 4 °C with constant agitation. Two hundred and fifty microlitres of beads were used per 250 × 10 6 cells. After washing with high-salt EB1000, FLAG-tagged MLE was eluted overnight at 4 °C with constant agitation in the presence of 0.5 mg ml −1 FLAG-Peptide (Sigma), concentrated (Amicon Ultra-4, Millipore) and rapidly frozen in liquid nitrogen. Protein concentrations were determined via SDS–PAGE and Coomassie staining using BSA (New England Biolabs) as a standard [24] . Chemical and enzymatic footprinting roX2 RNA (1.2 pmol) was resuspended in buffer D (20 mM Hepes-KOH pH 7.9, 100 mM KCl, 0.2 mM EDTA pH 7.9, 0.5 mM DTT, 0.5 mM PMSF, 20% (v/v) glycerol) to 80 nM concentration and renatured by heating at 65 °C for 10 min followed by slow cooling down to room temperature, with the addition of MgCl 2 to a final concentration of 6 mM and preincubation for 10 min at room temperature. RNA was incubated for 10 min at 30 °C with recombinant UNR (0.88, 1.75 and 3.5 μM). RNase T2 (0.25 U) was added under conditions such that a partial digestion of single-stranded segments was achieved. DMS (1 μl of a 1/60 (v/v) DMS/EtOH solution) was employed to modify single-stranded A and C residues. Reactions were stopped by ethanol precipitation. The RNA was washed with 70% ethanol and dissolved in 6 μl of water. One microlitre of this solution was used for a reverse transcriptase elongation assay allowing to detect cleavage and modification positions [25] . MS2-affinity chromatography MS2-tagged RNAs (5.6 pmol) were denatured by incubation at 65 °C for 5 min and renatured by slow cooling down to room temperature. Subsequently, the RNA was incubated with a 10-fold molar excess of purified MS2–MBP for 15 min at 4 °C. Then, the RNA–MS2–MBP complexes were incubated with 20 μl amylose resin (Bio-Rad; pre-equilibrated in buffer D) for 30 min at 4 °C. After three washes with 900 μl of buffer D, 4 to 40 nM of MLE and/or 80 nM of UNR in a total volume of 300 μl of buffer D supplemented with 5 μM yeast tRNA (Sigma), ATP (1 mM) and RNasin (Promega) were added. After 10 min of incubation at 25 °C with constant agitation, three successive washes with Buffer D were performed. RNPs were eluted with 40 μl buffer D containing 10 mM maltose for 15 min at 4 °C. Twenty-five % of the eluted material was used for western blot analysis using specific MLE or UNR antibodies. The RNA content of the eluted fractions was analysed on denaturing polyacrylamide gels stained with ethidium bromide. ChIP Male Drosophila S2 cells were cultured and crosslinked in growth medium using 1% formaldehyde for 60 min on iced water. Fixation was quenched by addition of glycine to a final concentration of 125 mM. After washing with PBS, cells were resuspended in RIPA buffer (1% Triton X-100, 0.1% Na deoxycholate, 0.1% SDS, 140 mM NaCl, 10 mM Tris pH 8.0, 1 mM EDTA) at a concentration of 1 × 10 7 cells per 100 μl. Eight hundred microlitres of crosslinked cells were sheared using Covaris S220 machine with a peak incident power of 100 W, duty factor 20%, 200 cycles/burst for 20 min to obtain 180-bp chromatin. Two hundred microlitres chromatin was precleared using 30 μl of a protein A/protein G-sepharose mixture for 1 h at 4 °C. For MLE-ChIP, after an incubation of 30 μl of protein A/protein G-sepharose mixture for 1 h at room temperature with 10 μg of anti-rat bridging antibody (Dianova) in a final volume of 500 μl RIPA buffer, MLE antibody was added and incubated for 4 h at 4 °C. This mix was washed with RIPA, and the precleared chromatin added, followed by overnight incubation at 4 °C. For MOF-ChIP, MOF antibody was incubated with the pre-cleared chromatin overnight at 4 °C. Complexes were purified by incubation for 3 h with 30 μl of a protein A/protein G-sepharose mixture. After washing and crosslink reversal, immunoprecipitated nucleic acids were purified on GenElute columns (Sigma). Input chromatin serving as reference sample was treated accordingly. Input material (10%) and eluted DNA were subjected to RT–qPCR with SYBR green (Applied Biosystems) using HAS or promoter-specific oligonucleotides [3] (detailed in Supplementary Table 1 ). Values were normalized to internal controls and to input. Differences between data sets in at least four independent experiments were tested for significance using the Student’s t -test, and P values lower than 0.05 were considered significant (* P <0.05; ** P <0.005; *** P <0.001). How to cite this article: Militti, C. et al. UNR facilitates the interaction of MLE with the lncRNA roX2 during Drosophila dosage compensation. Nat. Commun. 5:4762 doi: 10.1038/ncomms5762 (2014).